Enterobacteria-secreted particles induce production of exosome-like S1P-containing particles by intestinal epithelium to drive Th17-mediated tumorigenesis Gut-associated inflammation plays a crucial role in the progression of colon cancer. Here, we identify a novel pathogen–host interaction that promotes gut inflammation and the development of colon cancer. We find that enteropathogenic bacteria-secreted particles (ET-BSPs) stimulate intestinal epithelium to produce IDENs (intestinal mucosa-derived exosome-like nanoparticles) containing elevated levels of sphingosine-1-phosphate, CCL20 and prostaglandin E2 (PGE2). CCL20 and PGE2 are required for the recruitment and proliferation, respectively, of Th17 cells, and these processes also involve the MyD88-mediated pathway. By influencing the recruitment and proliferation of Th17 cells in the intestine, IDENs promote colon cancer. We demonstrate the biological effect of sphingosine-1-phosphate contained in IDENs on tumour growth in spontaneous and transplanted colon cancer mouse models. These findings provide deeper insights into how host–microbe relationships are mediated by particles secreted from both bacterial and host cells. Dysregulation of the interactions between the gut epithelium and intestinal bacteria leads to the loss of host immune tolerance and promotes the development of colon cancer [1] . The mechanism by which these interactions regulate host immune response during cancer progression has not been completely characterized. Recently, the tumorigenic function of exosomes has become widely recognized [2] , [3] . However, the potential role of intestinal mucosa-derived exosome-like nanoparticles (IDENs) [4] , [5] in the regulation of the intestinal immune system of a colon tumour-bearing host has not been studied. On the basis of the characteristics of exosomes released from intestinal epithelial cell (IEC) lines, it has been suggested that IEC-derived exosomes influence antigen presentation [6] and antimicrobial responses [7] . However, because cell culture cannot completely mimic the microenvironment of the gut community of a host bearing a colon tumour, it has not been possible to determine whether the exosomes in the intestinal mucosa of a colon tumour-bearing host regulate the host immune response by communicating with intestinal bacteria. We hypothesize that, along with epithelial cells, intestinal bacteria and immune cells, IDENs in the intestinal mucosa play a crucial role in gut immune regulation. As a proof of concept, we used three well-established Th17-regulated colon cancer mouse models to determine whether IDENs under different pathophysiological conditions play a role in the induction of intestinal Th17 cells by communicating with enterobacteria (ET)-secreted particles (ET-BSPs). In particular, we investigated whether IDENs contribute to the development of Th17-mediated colon tumours and whether the biological functions of IDENs can be altered through interactions with intestinal bacteria. In this study, we find that sphingosine-1-phosphate (S1P) contained by IDENs mediates their effects and lead to the promotion of tumour growth through the induction of Th17 cells. The enrichment of IDENs with S1P is induced by ET-BSPs ( Fig. 1a ). The intestinal macrophage PGE2 induced by IDEN CCL20+PGE2+ S1P+ further drives the overproduction of CD4 + CCR6 + IL17A + cells in colon tumour-bearing hosts ( Fig. 1b ). Using APC Min/+ mice and MyD88 −/− or APC Min/+ MyD88 −/− mouse tumour models, we further demonstrate that the MyD88-mediated pathway plays a role in the APC Min/+ IDEN (APC-IDEN)-mediated recruitment and activation of CCR6 + CD4 + Th17 + cells. Collectively, IDENs communicate with the established mammalian gut community and regulate gut immune homeostasis. Dysregulation of the composition of IDENs (for example, the overproduction of S1P) promotes colon tumour growth. 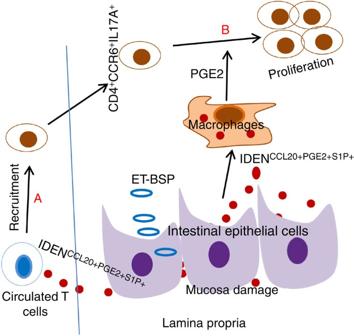Figure 1: Proposed pathways lead to overproduction of CD4+CCR6+IL17A+. (a) ET-BSP uptake by intestinal epithelial cells leads to induction of IDENCCL20+PGE2+S1P+. Owing to increasing gut permeability or mucosa damage, released IDENCCL20+PGE2+SIP+subsequently migrate into the peripheral blood and induce CCR6 expression on CD4 T cells, which results in more CD4+CCR6+IL17A+cells being recruited into intestinal tissue. (b) Uptake of IDENCCL20+PGE2+S1P+by intestinal macrophages results in induction of PGE2, which then promotes more production of CD4+CCR6+IL17A+. Figure 1: Proposed pathways lead to overproduction of CD4 + CCR6 + IL17A + . ( a ) ET-BSP uptake by intestinal epithelial cells leads to induction of IDEN CCL20+PGE2+S1P+ . Owing to increasing gut permeability or mucosa damage, released IDEN CCL20+PGE2+SIP+ subsequently migrate into the peripheral blood and induce CCR6 expression on CD4 T cells, which results in more CD4 + CCR6 + IL17A + cells being recruited into intestinal tissue. ( b ) Uptake of IDEN CCL20+PGE2+S1P+ by intestinal macrophages results in induction of PGE2, which then promotes more production of CD4 + CCR6 + IL17A + . Full size image Uptake of ET-BSPs by IECs leads to the induction of Th17 cells Increasing the number of CD4 + Th17 + cells in animal models of colorectal cancer has been demonstrated to have procarcinogenic effects [8] , [9] , [10] . Published data [11] suggest that ETBF (enterotoxigenic Bacteroides fragilis ) helps to induce the Th17-cell-mediated promotion of colon carcinogenesis. The mechanism by which Th17 cells are induced by ETBF is not completely understood. To investigate the role of ET-BSPs (here used to refer to ET-BSPs from enterotoxigenic Bacteroides fragilis ) in the induction of Th17 cells and colon inflammation, mice were given drinking water containing 2.5% DSS to induce colitis and were then treated with ET-BSPs. ET-BSPs accelerated the loss of body weight and reduction of colon length in mice with DSS-induced colitis ( Supplementary Fig. S1a,b ). When administered orally to DSS-treated mice, BSPs derived from nontoxigenic B. fragilis (henceforth referred to as ‘NT-BSPs’) offered significant protection against weight loss and reduction of colon length ( Supplementary Fig. S1a,b ), consistent with results by others [12] , [13] . Interestingly, NT-BSPs induce Foxp3 + CD4 + T cells, whereas ET-BSPs induce the accumulation of CD4 + IL-17A + cells in the colon ( Supplementary Fig. S1c ). To identify which types of intestinal cells take up BSPs, we gavaged colitic mice with BSPs labelled with PKH26 dye. The resulting colon section images show that BSPs are associated with intestinal epithelial cells and macrophages ( Supplementary Fig. S2 ). The biological effects of ET-BSPs on the recipient cells were further investigated both in vitro and in vivo . ET-BSPs increased the expression of CCL20, COX-2 and genes encoding proinflammatory molecules in macrophages (that is, IL-6, IL-23, TNF-α and MMP9) ( Supplementary Fig. S3 ). To determine whether macrophages exposed to ET-BSPs play a role in the induction of CD4 + Th17 + cells, OT-II naive CD4 + T cells were cultured with colonic macrophages treated with ET-BSPs or NT-BSPs in the presence of OVA. NT-BSP-treated macrophages induced the expression of IL-10 in macrophage T-cell co-cultures, whereas minimal IL-10 was detected in co-cultures of ET-BSP-treated macrophages and CD4 + T cells. However, co-cultures of ET-BSP-treated macrophages and CD4 + T cells had higher quantities of IL-17A and IL-6 in their culture supernatants compared with NT-BSP-treated macrophage/CD4 + T-cell co-cultures ( Supplementary Fig. S4a ). The results of real-time PCR showed that CD4 + Th17 + cells co-cultured with ET-BSP-treated macrophages contained higher levels of IL-17A, IFN-γ, IL-6 and the T-cell homing markers CCR6 and CCR9 than did CD4 + Th17 + cells co-cultured with NT-BSP-treated macrophages, but lower levels of IL-10 and IL-4 ( Supplementary Fig. S4b ). Next, we treated mice with ET-BSPs or NT-BSPs by daily colonic submucosal injection for 10 days. After this period, we observed extensive accumulation of CD4 + IL-17A + cells and F4/80 + macrophages in the colon ( Supplementary Fig. S4c ). To determine the molecular basis of this ET-BSP-mediated production of Th17 cells, the mice were treated by colonic submucosal injection of bacterial secreted particles from NTBFs genetically engineered to produce B. fragilis toxin (γETBF) [11] . Injection of BSPs from γETBF led to the detection of a higher percentage of Th17 cells at the injection sites when compared with mice that received wild-type NT-BSPs from WT-NTBF ( Supplementary Fig. S4d , top panel). Furthermore, treatment with BSPs from NTBFs expressing a mutation of the B. fragilis toxin gene (ΔBFT) [11] did not lead to an increase in Th17 cells. Collectively, these results suggest that the B. fragilis toxin gene plays a role in the ET-BSP-mediated proliferation of Th17 cells. Using a similar approach, we also showed that polysaccharide A ( PSA) from wild-type NT-BSP bacteria [14] plays a role in the NT-BSP–mediated induction of Foxp3 ( Supplementary Fig. S4d , middle panel). Innate lymphoid cells (ILCs) also contribute to gut homeostasis. No significant difference was detected in the accumulation of IL-22 + ILCs in the colons of naive mice injected with BSPs from γETBF when compared with naive mice injected with BSPs from ΔBFT ( Supplementary Fig. S4d , the bottom panel), suggesting that the B. fragilis toxin protein preferentially regulates the induction of inflammatory cells. To further determine the biological effects of ET-BSPs on epithelial cells, we examined gene expression in MC38 colon cells incubated with either NT-BSPs or ET-BSPs. Real-time PCR analysis showed that CCL20, CCL4, CXCL9 and COX2 were induced in MC38 cells stimulated with ET-BSPs but not NT-BSPs ( Supplementary Fig. S5 ). The expression of SphK1 was elevated significantly in MC38 cells treated with ET-BSPs compared with those treated with NT-BSPs ( Fig. 2a ). SphK1 is an enzyme that catalyses the synthesis of S1P. The S1P has been implicated in the induction of several inflammatory mediators, including PGE2. We next investigated the effect of S1P on the production of PGE2 in primary cultured intestinal epithelial cells. As shown in Fig. 2b , S1P promotes the expression of numerous chemokine genes as well as COX2, SphK1 and Sphk2. In addition, the induction of COX2 was consistent with the increase in PGE2 after S1P stimulation. As ET-BSPs can also be taken up by intestinal macrophages, MC38 cells were incubated with the supernatant from colonic macrophages stimulated with ET-BSPs or NT-BSPs. SphK1, SphK2 and COX2 were induced in MC38 cells treated with conditioned medium (CM) from ET-BSP-stimulated macrophages (ET-BSP-CM), but not from NT-BSP-stimulated macrophages (NT-BSP-CM) ( Fig. 2c ). Together, our data suggest that ET-BSPs induce the expression of Sphk1 and PGE2 in intestinal epithelial cells. 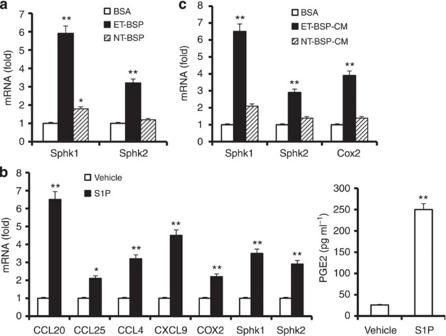Figure 2: ET-BSPs and S1P upregulate genes that encode sphingolipids and chemokines. Molecules expressed in MC38 cells (a,b). MC38 colon cancer cells were cultured with BSA, NT-BSPs or ET-BSPs (20 μg ml−1) (a) or with vehicle/S1P (b) for 18 h. Real-time PCR analysis of gene expression (a,b, left panel) and ELISA analysis of PGE2 (right panel) in the supernatants. The data represent means±s.e.m. *P<0.05,**P<0.01 (Student’st-test). (c) MC38 cells were cultured with conditioned medium from colonic macrophages treated with BSA, NT-BSPs or ET-BSPs, and the expression of the indicated genes was measured by qPCR. The data represent means±s.e.m. (n=5). *P<0.05,**P<0.01 (Student’st-test). Figure 2: ET-BSPs and S1P upregulate genes that encode sphingolipids and chemokines. Molecules expressed in MC38 cells ( a , b ). MC38 colon cancer cells were cultured with BSA, NT-BSPs or ET-BSPs (20 μg ml −1 ) ( a ) or with vehicle/S1P ( b ) for 18 h. Real-time PCR analysis of gene expression ( a , b , left panel) and ELISA analysis of PGE2 (right panel) in the supernatants. The data represent means±s.e.m. * P <0.05, ** P <0.01 (Student’s t -test). ( c ) MC38 cells were cultured with conditioned medium from colonic macrophages treated with BSA, NT-BSPs or ET-BSPs, and the expression of the indicated genes was measured by qPCR. The data represent means±s.e.m. ( n =5). * P <0.05, ** P <0.01 (Student’s t -test). Full size image The uptake of ET-BSPs leads to an overproduction of exosomal S1P On the basis of results presented above, we hypothesized that intestinal bacteria regulate IDEN composition and subsequently have an effect on the induction of Th17 cells by ET-BSPs. An analysis of exosomes (IDENs that are isolated and purified from the supernatant of a cultured cell line such as MC38) derived from MC38 cells stimulated with ET-BSP-CM showed high levels of SPH, which is a substrate of Sphk1 used in the synthesis of S1P ( Fig. 3a ) and CCL20 ( Fig. 3b ). CCL20 is a ligand for the recruitment of CCR6 + Th17 cells. We investigated whether S1P is induced after ET-BSP stimulation and leads to enrichment of S1P in exosomes. Exosomes were sucrose-purified from the supernatants of MC38 cells co-cultured for 48 h with ET-BSPs or NT-BSPs (named ET-Tumour EXO and NT-Tumour EXO , respectively); BSA served as a control (BSA-Tumour EXO ). ET-Tumour EXO contained higher levels of PGE2 and S1P than NT-Tumour EXO or BSA-Tumour EXO ( Fig. 3c ). Ceramide is involved in exosome biogenesis [15] and can be metabolized by ceramidase to sphingosine (SPH), which can be metabolized in turn to S1P by sphingosine kinase (SphK1). To determine whether SphK1 is involved in the induction of exosomal S1P, MC38 cells were treated with an SphK1 inhibitor (SK1-I) in the presence of ET-BSPs. As expected, the levels of S1P in ET-Tumour EXO decreased significantly after SK1-I treatment ( Fig. 3c ). Interestingly, exosomal PGE2 ( Fig. 3c ) and CCL20 ( Fig. 3d ) were also downregulated by SKI-1. Collectively, these data suggest that ET-BSPs induce exosomal S1P, which further enhances the production of CCL20 + PGE2 + S1P + exosomes. 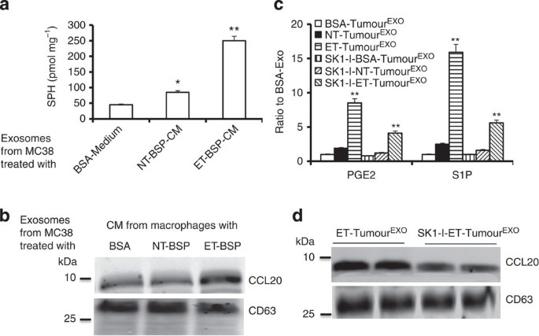Figure 3: Bacteria-secreted particles mediate the induction of CCL20+PGE2+S1P+exosomes. (a,b) MC38 cells were cultured with conditioned medium (CM) from macrophages treated with BSA, NT-BSPs or ET-BSPs (20 μg ml−1), and the levels of SPH (a) and CCL20 (b) in tumour exosomes were assessed by LC-MS/MS (a) or western blot (b). The data represent means±SEMs (n=5). *P<0.05,**P<0.01 (Student’st-test). (c) Changes in the ratio of S1P and PGE2 in exosomes released from MC38 cells pretreated with BSA, NT-BSPs or ET-BSPs in the absence or presence of SphK1 inhibitor (SK1-I, 5 μM ) for 48 h. The data represent means±s.e.m..**P<0.01 (Student’st-test). (d) Western blot analysis of CCL20 in exosomes derived from (c). Figure 3: Bacteria-secreted particles mediate the induction of CCL20 + PGE2 + S1P + exosomes. ( a , b ) MC38 cells were cultured with conditioned medium (CM) from macrophages treated with BSA, NT-BSPs or ET-BSPs (20 μg ml −1 ), and the levels of SPH ( a ) and CCL20 ( b ) in tumour exosomes were assessed by LC-MS/MS ( a ) or western blot ( b ). The data represent means±SEMs ( n =5). * P <0.05, ** P <0.01 (Student’s t -test). ( c ) Changes in the ratio of S1P and PGE2 in exosomes released from MC38 cells pretreated with BSA, NT-BSPs or ET-BSPs in the absence or presence of SphK1 inhibitor (SK1-I, 5 μM ) for 48 h. The data represent means±s.e.m.. ** P <0.01 (Student’s t -test). ( d ) Western blot analysis of CCL20 in exosomes derived from ( c ). Full size image ET-Tumour EXO S1P-activated Stat3 promotes tumour growth To explore whether ET-Tumour EXO could contribute to the promotion of colon cancer, we implanted MC38 tumours with ET-Tumour EXO or NT-Tumour EXO by orthotropic colonic submucosal microinjection. Co-injection of ET-Tumour EXO markedly promoted MC38 tumour growth compared with NT-Tumour EXO ( Fig. 4a–c ), which further prompted us to analyse whether S1P + -enriched ET-Tumour EXO could participate in promoting the progression of colon cancer via the induction of CD4 + Th17 + . FACS analysis indicated that there were significantly more CD4 + IL-17A + cells in the tumours harvested from mice treated with ET-Tumour EXO than those treated with NT-Tumour EXO ( Fig. 4d ). By contrast, mice treated with NT-Tumour EXO had a high percentage of FoxP3 + Tregs ( Fig. 4d ). The quantity of IL-17A-producing CD8 + cells was also increased two- to threefold in tumours from ET-Tumour EXO -treated mice compared with NT-Tumour EXO -treated mice ( Supplementary Fig. S6a ). Real-time PCR results confirmed that IL-17A and CCR6 mRNA, but not IL-10 mRNA, were increased in tumours from ET-Tumour EXO -treated mice compared with NT-Tumour EXO -treated mice ( Fig. 4e ). Furthermore, higher percentages of TNFα-producing CD4 + T cells and IFN-γ-producing Th1 cells were observed in the ET-Tumour EXO -treated mice ( Supplementary Fig. S6b ). 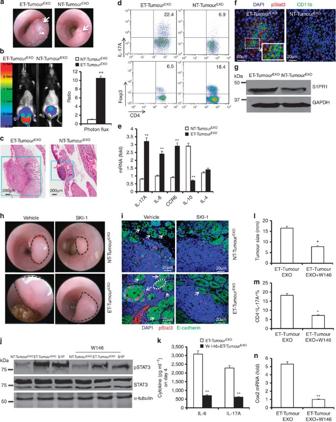Figure 4: ET-TumourEXOaccelerates tumour growth by modulating Stat3 signalling. (a–c) C57BL/6 mice were orthotopically implanted with MC38-luc cells with exosomes by colonic submucosal injection. Colonoscopy image of implanted MC38-luc cells at day 18 after injection (a), photon flux from C57BL/6 mice harbouring MC38-luc tumours (b) and H&E-stained colon sections (c). The data (b) represent means±s.e.m.**P<0.01 (Student’st-test). (d) Colonic MC38 tumour leukocytes were isolated at day 18 post treatment from mice treated with ET-TumourEXOor NT-TumourEXO. TCRβ+CD4+IL-17A+and FoxP3+Treg cell populations were examined by FACS. (e) RT-PCR analysis of the gene expression in colonic MC38 tumour leukocytes isolated at day 18 from mice treated with ET-TumourEXOor NT-TumourEXO. (f,g) Confocal images of colon sections stained with p-Stat3 and CD11b from naive mice treated with ET-TumourEXOor NT-TumourEXO(f); western blotting the lysates of colonic CD11b+cells for S1PR1 (g). (h,i) Mice were orthotopically implanted with MC38 cells mixed with exosomes from MC38 cells with or without SK1-I. Colonoscopy image of MC38 tumour size (h); confocal images of colon sections stained with p-Stat3 and E-cadherin (i). (j) Western blotting showing p-Stat3 proteins in LPLs stimulated by anti-CD3 (5 μg ml−1) and CD28 (2 μg ml−1) antibodies in the presence of NT-TumourEXO, ET-TumourEXO(50 μg ml−1) or S1P (100 nM) with or without W146 (20 nM) for 24 h. (k) ELISA analysis of IL-6 and IL-17A in the supernatants of LPLs stimulated with anti-CD3 and CD28 antibodies in the presence of ET-TumourEXO(50 μg ml−1) with or without W146 (20 nM) after 4 days in culture. (l–n) Mice were orthotopically implanted with MC38 cells mixed with ET-tumour exosomes and treated with or without W146. Tumour size (l), number of CD4+IL-17A+cells in the colon (n), expression of COX2 in the colon (n). The data (e,k–n) represent means±s.e.m. (n=5). *P<0.05,**P<0.01 (Student’st-test). Figure 4: ET-Tumour EXO accelerates tumour growth by modulating Stat3 signalling. ( a – c ) C57BL/6 mice were orthotopically implanted with MC38-luc cells with exosomes by colonic submucosal injection. Colonoscopy image of implanted MC38-luc cells at day 18 after injection ( a ), photon flux from C57BL/6 mice harbouring MC38-luc tumours ( b ) and H&E-stained colon sections ( c ). The data ( b ) represent means±s.e.m. ** P <0.01 (Student’s t -test). ( d ) Colonic MC38 tumour leukocytes were isolated at day 18 post treatment from mice treated with ET-Tumour EXO or NT-Tumour EXO . TCRβ + CD4 + IL-17A + and FoxP3 + Treg cell populations were examined by FACS. ( e ) RT-PCR analysis of the gene expression in colonic MC38 tumour leukocytes isolated at day 18 from mice treated with ET-Tumour EXO or NT-Tumour EXO . ( f , g ) Confocal images of colon sections stained with p-Stat3 and CD11b from naive mice treated with ET-Tumour EXO or NT-Tumour EXO ( f ); western blotting the lysates of colonic CD11b + cells for S1PR1 ( g ). ( h , i ) Mice were orthotopically implanted with MC38 cells mixed with exosomes from MC38 cells with or without SK1-I. Colonoscopy image of MC38 tumour size ( h ); confocal images of colon sections stained with p-Stat3 and E-cadherin ( i ). ( j ) Western blotting showing p-Stat3 proteins in LPLs stimulated by anti-CD3 (5 μg ml −1 ) and CD28 (2 μg ml −1 ) antibodies in the presence of NT-Tumour EXO , ET-Tumour EXO (50 μg ml −1 ) or S1P (100 nM) with or without W146 (20 nM) for 24 h. ( k ) ELISA analysis of IL-6 and IL-17A in the supernatants of LPLs stimulated with anti-CD3 and CD28 antibodies in the presence of ET-Tumour EXO (50 μg ml −1 ) with or without W146 (20 nM) after 4 days in culture. ( l – n ) Mice were orthotopically implanted with MC38 cells mixed with ET-tumour exosomes and treated with or without W146. Tumour size ( l ), number of CD4 + IL-17A + cells in the colon ( n ), expression of COX2 in the colon ( n ). The data ( e , k – n ) represent means±s.e.m. ( n =5). * P <0.05, ** P <0.01 (Student’s t -test). Full size image A recent study suggests that sphingosine kinase-1 (SphK1), which is highly elevated in tumours, is regulated by S1PR1-STAT3 signalling [16] . We therefore investigated whether blocking SIP production had similar effects as ET-Tumour EXO on the induction of IL-17A and IL-6 by treating exosome-producing cells with SK1-I. SK1-I-ET-Tumour EXO or ET-Tumour EXO was added to cultures of OT-II CD4 T cells in the presence of OVA peptide and colonic macrophages. Analysis of the culture supernatants showed a reduction in inflammatory cytokines, particularly IL-6 and IL-17A ( Supplementary Fig. S7 ), in the cells treated with SK1-I-ET-Tumour EXO in comparison with ET-Tumour EXO . Previously published data suggest that the S1P-mediated pathway might activate Stat3 (refs 16 , 17 ) and that many different cells express S1P receptors. We found that naive mice treated with ET-Tumour EXO had an extensive accumulation of CD11b + myeloid cells in their intestinal tissue and widespread Stat3 activation and S1PR1 expression on myeloid cells ( Fig. 4f,g ). Furthermore, SK1-I-ET-Tumour EXO was markedly less effective than ET-Tumour EXO in promoting MC38 tumour growth ( Fig. 4h ), as evidenced by a decrease in proliferating epithelial cells, that is, Ki-67 + cells ( Supplementary Fig. S8 ). Importantly, the phosphorylation of Stat3 was significantly decreased in the epithelium after SK1-I-ET-Tumour EXO treatment ( Fig. 4i ). The role of S1PR1-STAT3 signalling was supported by a significant decrease in STAT3 phosphorylation after treatment with W146, a competitive S1PR1 antagonist ( Fig. 4j ). We also found that W146 significantly decreased IL-17A and IL-6 secretion in LPLs treated with ET-Tumour EXO ( Fig. 4k ). The results from an in vivo study also support the idea that W146 suppresses ET-Tumour EXO -induced tumour growth, the reduction in colonic CD4 + IL-17A + cells and the expression of COX2 in MC38 tumour-bearing mice ( Fig. 4l–n ). CCR6 + CD4 + Th17 + cells induced by APC-IDENs promote tumour growth A challenging question in exosome biology is whether the biological effects of cell culture-derived exosomes can mimic those of endogenous exosomes isolated in vivo . APC Min/+ mice were used to address whether exosomes isolated from the intestinal mucosa of mice under physiological and pathophysiological conditions play similar roles to exosomes from the MC38 cell line. APC Min/+ is a point mutation in the murine homologue of the APC gene [18] . APC Min/+ mice develop multiple intestinal adenomas, as do humans carrying germ-line mutations in APC. Our previously published data indicated that numerous IDEN particles accumulate in the intestinal mucosa and help to regulate gut immune function [4] , [5] . In the present study, an increase in S1P was confirmed in the circulating exosomes and IDENs of APC Min/+ , CAC and DSS mice ( Supplementary Fig. S9a ). Sphingosine was also elevated in the circulating exosomes and IDENs of APC Min/+ , CAC and DSS mice when compared with WT mice ( Supplementary Fig. S9b ). To investigate whether APC-IDENs play a role similar to that of MC38 tumour exosomes in terms of tumour progression, APC Min/+ female mice were gavaged with APC-IDENs or WT-IDENs as a control every 3 days for 8 weeks. Treatment with APC-IDENs ( Fig. 5a ) resulted in increased tumour incidence and size compared with WT-IDEN treatment. The results in the mouse APC min/+ tumour model were repeated in an azoxymethane/DSS (AOM/DSS) tumour model ( Supplementary Fig. S10 ). Histological examination of the small intestine showed a marked enhancement of the proliferation of IECs after APC-IDEN treatment, as measured by BrdU incorporation ( Fig. 5b ). The phosphorylation of epithelial STAT3 and ERK1/2, both of which have roles in promoting colon cancer progression, was also found to be increased after APC-IDEN treatment ( Fig. 5c ). FACS analysis showed that the quantity of CCR6 + CD4 + T cells was significantly increased in the tumours of mice treated with APC-IDENs ( Supplementary Fig. S11a ) or CAC-IDENs ( Supplementary Fig. S11b ) in comparison with WT-IDENs. Furthermore, FACS analysis identified a higher percentage of intestinal CCR6 + CD4 + Th17 + cells in mice treated with APC-IDENs compared with those treated with WT-IDENs ( Fig. 5d ). Real-time PCR analysis showed that expression of IL-17A and IL-6 was higher in colonic CD4 + T cells from mice treated with APC-IDENs compared with WT-IDENs ( Fig. 5d ). To assess whether the increase in IL-17A contributed to tumorigenesis, IL-17A was neutralized with an IP injection of anti-mouse IL-17A antibodies in APC-IDEN–treated APC Min/+ mice. The results, including colonic inflammation, proliferation of epithelial cells and tumour numbers ( Fig. 5e–g ), suggest that the neutralization of IL-17A eliminates the tumorigenic effects of APC-IDENs. 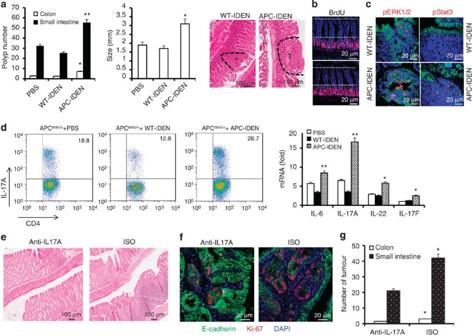Figure 5: APC-IDENs promote tumour growth by inducing CCR6+CD4+Th17+cells. (a–c) APCmin/+mice at 6 weeks of age were gavaged with IDENs once every 3 days for 8 weeks. (a) Number and size of tumours and H&E-stained sections from 3-month-old APCMin/+mice. (b) Mice were injected intraperitoneally (i.p.) with 50 mg kg−1of 5’-bromo-2’-deoxyuridine (BrdU) in PBS 24 h before small intestine harvest. BrdU antibody-stained small intestine sections. (c) A sectioned tumour was stained with an anti-phospho-ERK antibody (red) or phospho-STAT3 (red) and E-cadherin (green). The data (a) represent means±s.e.m. (n=8). *P<0.05,**P<0.01 (Student’st-test). (d) FACS analysis of IL-17A+on CCR6+CD4+T cells and real-time PCR for cytokine mRNAs in LPL CCR6+CD4+T cells. The data represent means±s.e.m. (n=5). *P<0.05,**P<0.01 (Student’st-test). (e–g) APCmin/+mice gavaged with IDENs were treated with an anti-IL17A antibody or isotype. Representative photomicrographs of HE-stained colon sections (e), immunofluorescent staining of colon sections with anti-E-cadherin and Ki67 (f), and number of tumours (g). Figure 5: APC-IDENs promote tumour growth by inducing CCR6 + CD4 + Th17 + cells. ( a – c ) APC min/+ mice at 6 weeks of age were gavaged with IDENs once every 3 days for 8 weeks. ( a ) Number and size of tumours and H&E-stained sections from 3-month-old APC Min/+ mice. ( b ) Mice were injected intraperitoneally (i.p.) with 50 mg kg −1 of 5’-bromo-2’-deoxyuridine (BrdU) in PBS 24 h before small intestine harvest. BrdU antibody-stained small intestine sections. ( c ) A sectioned tumour was stained with an anti-phospho-ERK antibody (red) or phospho-STAT3 (red) and E-cadherin (green). The data ( a ) represent means±s.e.m. ( n =8). * P <0.05, ** P <0.01 (Student’s t -test). ( d ) FACS analysis of IL-17A + on CCR6 + CD4 + T cells and real-time PCR for cytokine mRNAs in LPL CCR6 + CD4 + T cells. The data represent means±s.e.m. ( n =5). * P <0.05, ** P <0.01 (Student’s t -test). ( e – g ) APC min/+ mice gavaged with IDENs were treated with an anti-IL17A antibody or isotype. Representative photomicrographs of HE-stained colon sections ( e ), immunofluorescent staining of colon sections with anti-E-cadherin and Ki67 ( f ), and number of tumours ( g ). Full size image APC-IDENs induce CCR6 + CD4 + Th17 + cell homing to the gut Our data showed that (1) double PKH26 + F4/80 + fluorescence increased in the lamina propria of the large intestines of APC Min/+ mice ( Fig. 6a ); (2) PKH26-labelled IDENs were also evident in the tumours of APC Min/+ mice ( Fig. 6b ); and (3) macrophages from small intestinal lamina propria (SI-LP) captured PKH26-labelled IDENs bound to GFP-bacteria and the captured IDENs were present in macrophages F4/80+ ( Fig. 6c , left panel). In comparison with WT-IDENs, colonic macrophages that were cultured in the presence of APC-IDENs and intestinal bacterial lysates secreted higher levels of CCL20 ( Fig. 6d ). APC-IDENs also increased the production of IL-23, IL-6 and TNF-α. Thus, the uptake of APC-IDENs by macrophages (macrophages APC-IDEN+ ) leads to the induction of CCL20, which is a specific ligand for recruiting CCR6 + CD4 + Th17 + cells. Western blot analysis indicates that the levels of CCL20 are much higher in IDENs from APC min/+ and CAC mice than in those from WT mice ( Fig. 6e ). Collectively, macrophages APC-IDEN+ and APC-IDENs provide a CCL20-enriched source for the possible recruitment of CCR6 + CD4 + Th17 + T cells into the intestine. 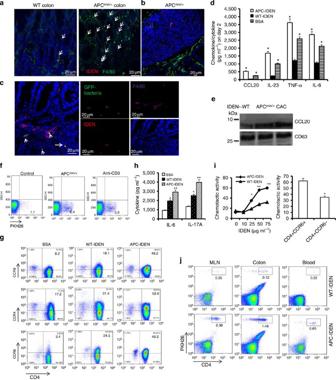Figure 6: APC-IDENs and macrophageAPC-IDEN+recruit CCR6+CD4+Th17+to the gut. (a–c) Confocal images of F4/80 immuno-stained frozen colon sections prepared 5 h after gavaging mice with PKH26-labelled IDENs (red). Non-tumour (a) and tumour (b) colon sections from APCmin/+mice. (c) Confocal images of the co-localization of macrophages (purple), IDENs (red) and bacteria (green) in SI tissue sections from APCmin/+mice gavaged with IDENs and bacteria tagged with GFP. (d) ELISA analysis of CCL20, IL-23, TNF-α and IL-6 in the supernatants of macrophages cultured for 2 days in the presence of bacterial lysate and WT-IDENs, APC-IDENs or BSA. (e) Western blot analysis of IDEN CCL20 from normal (WT), APCmin/+or CAC mice. (f) FACS analysis of PKH26+cells in peripheral blood from naive mice, APCmin/+mice or anti-CD3-treated mice after gavage with PKH26-labelled IDENs. (g) Chemokine receptors induced on naive CD4+T cells under Th17+cell culture conditions in the presence of BSA or IDENs. (h) ELISA analysis of IL-6 and IL-17A in the supernatants from (g). (i) Chemotactic responses of APCmin/+mouse CD4+T cells to IDENs (left) or the migration of CCR6+/+versus CCR6−/−CD4+T cells to APC-IDENs (right)in vitro. (j) CD4+T cells cultured under Th17+cell culture conditions in the presence of IDENs were labelled with PKH26 and adoptively transferred intravenously into DSS-treated SCID mice. The cells were then isolated from the MLN, colon and blood for the FACS analysis of PKH26+CD4+T cells. The data (d,h,i) represent means±s.e.m. (n=5). *P<0.05,**P<0.01 (Student’st-test). Figure 6: APC-IDENs and macrophage APC-IDEN+ recruit CCR6 + CD4 + Th17 + to the gut. ( a – c ) Confocal images of F4/80 immuno-stained frozen colon sections prepared 5 h after gavaging mice with PKH26-labelled IDENs (red). Non-tumour ( a ) and tumour ( b ) colon sections from APC min/+ mice. ( c ) Confocal images of the co-localization of macrophages (purple), IDENs (red) and bacteria (green) in SI tissue sections from APC min/+ mice gavaged with IDENs and bacteria tagged with GFP. ( d ) ELISA analysis of CCL20, IL-23, TNF-α and IL-6 in the supernatants of macrophages cultured for 2 days in the presence of bacterial lysate and WT-IDENs, APC-IDENs or BSA. ( e ) Western blot analysis of IDEN CCL20 from normal (WT), APC min/+ or CAC mice. ( f ) FACS analysis of PKH26 + cells in peripheral blood from naive mice, APC min/+ mice or anti-CD3-treated mice after gavage with PKH26-labelled IDENs. ( g ) Chemokine receptors induced on naive CD4 + T cells under Th17 + cell culture conditions in the presence of BSA or IDENs. ( h ) ELISA analysis of IL-6 and IL-17A in the supernatants from ( g ). ( i ) Chemotactic responses of APC min/+ mouse CD4 + T cells to IDENs (left) or the migration of CCR6 +/+ versus CCR6 −/− CD4 + T cells to APC-IDENs (right) in vitro . ( j ) CD4 + T cells cultured under Th17 + cell culture conditions in the presence of IDENs were labelled with PKH26 and adoptively transferred intravenously into DSS-treated SCID mice. The cells were then isolated from the MLN, colon and blood for the FACS analysis of PKH26 + CD4 + T cells. The data ( d , h , i ) represent means±s.e.m. ( n =5). * P <0.05, ** P <0.01 (Student’s t -test). Full size image The induction of CCR6 expression on naive CD4 T cells is required to achieve preferential recruitment of Th17 cells to the gut [1] . FACS analysis indicated that a greater number of PKH26-labelled IDENs were circulating in the peripheral blood of APC Min/+ diseased mice than of naive mice after IDENs were given orally ( Fig. 6f ), suggesting that a higher quantity of IDENs are in circulation in the peripheral blood under pathophysiological conditions than under normal conditions. MUC2 is fundamental for maintaining the integrity of the intestinal barrier [19] , and CD3-specific antibody treatment induces intestinal inflammation, increases gut permeability [20] and promotes Th17-cell recruitment to the intestine [1] . Our FACS data indicate that higher levels of IDENs were in circulation in the peripheral blood of anti-CD3-treated mice than in that of naive control mice ( Fig. 6f ). This result was also consistent with the immunostaining of intestinal MUC2, indicating that mice that were pretreated with anti-CD3 antibodies exhibited a considerably lower level of intestinal MUC2 staining than those pretreated with a control IgG ( Supplementary Fig. S12a ). Next, we tested whether APC-IDEN treatment leads to an increase in molecules that encourage recruitment of Th17 cells to the gut such as CCR6, CCR4, CCR9, IL-6 and IL-17A. Our FACS analysis data indicate that CCR6, CCR4 and CCR9 expression on cultured T cells treated with APC-IDENs was much higher than on those treated with WT-IDENs ( Fig. 6g ). The supernatants from cultured T cells treated with APC-IDENs contained higher levels of inflammatory molecules, that is, IL-6 and IL-17A, than supernatants from WT-IDEN-treated cells ( Fig. 6h ). In accordance with the enhanced expression of these molecules, APC-IDEN treatment induced a stronger chemotactic activity in CD4 + T cells ( Fig. 6i ), partly through an increase in CCR6, which was demonstrated in CD4 + T cells from CCR6-KO mice ( Fig. 6i , right panel). APC-IDEN treatment leading to the enhanced expression of these molecules was also demonstrated in a co-culture of T-cell OVA pulsed macrophages ( Supplementary Fig. S12b ). The roles of APC-IDENs were further demonstrated with recruitment experiments in vivo . Equivalent numbers of PKH26-labelled naive CD4 + T cells were pretreated with WT-IDENs or APC-IDENs and adoptively transferred into recipients with DSS-induced colitis. CD4 + T cells treated with APC-IDENs induced greater migration of CD4 + cells from the blood into the inflamed colons of DSS-treated SCID mice than did CD4 + T cells treated with WT-IDENs ( Fig. 6j ). Furthermore, RAG1 −/− mice that received adoptively transferred CD4 + CD25 − CD62L hi naive T cells and were subsequently gavaged with APC-IDENs developed rapid and very severe colitis 7 weeks after the cell transfer, whereas mice who were gavaged with WT-IDENs did not. The exacerbation of colitis in the mice that received APC-IDENs was evidenced by greater weight loss, an accumulation of CD4 + Th17 + T cells and severe damage to epithelial cells, as indicated by severe dysplastic changes in the colon ( Supplementary Fig. S13a–13d ). Together, these data suggest that APC-IDENs have a direct effect on increasing the susceptibility of mice to colitis and carcinogenesis through the induction of inflammatory CCR6 + CD4 + Th17 + cell circulation and subsequent recruitment to the gut. APC-IDEN PGE2 plays a role in the accumulation of Th17 cells Our previously published data [4] , [21] suggest that exosomal PGE2 plays a role in immunomodulation. PGE2 is known to enhance the proliferation of CCR6 + Th17 + cells and the expression of CCL20 [22] . ELISA analysis indicated that the level of PGE2 was much higher in the IDENs from APC min/+ and CAC mice than from those from naive WT mice ( Fig. 7a ). The induction of IDEN PGE2 was not only demonstrated in the tumour models we tested but also in an anti-CD3 induced inflammation mouse model. Anti-CD3 treatment significantly increased COX2 expression in WT mice, and increased levels of PGE2 were detected in their IDENs ( Fig. 7b ). To confirm that PGE2/COX2 signalling was involved in Th17 accumulation in the intestine, mice treated with the COX2 inhibitors indomethacin and celecoxib during anti-CD3 treatment showed a noticeable decrease in accumulation of CD4 + IL-17A + cells ( Fig. 7c and Supplementary Fig. S14a ) and liquid stool ( Supplementary Fig. S14b ) in the small intestine. A recent study showed that Th17-cell expansion induced by PGE2 is mediated by EP4 (ref. 23 ). Consistent with these results, naive T cells were activated when they were cultured with APC-IDENs, and there was a significant increase in IL-17A production in cells cultured with APC-IDENs when compared with WT-IDENs ( Fig. 7d ). AH6809 (an EP2-selective antagonist) and ONO-AE3–208 (an EP4-selective antagonist) partially reversed APC-IDEN PGE2-induced IL-17A production ( Fig. 7d ). 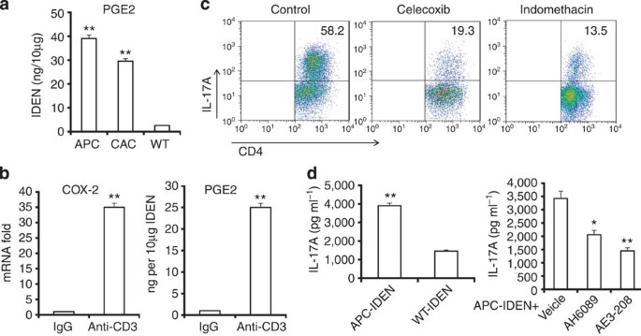Figure 7: APC-IDEN PGE2 plays a role in the accumulation of intestinal CD4+Th17+cells. (a) ELISA analysis of PGE2 in IDENs isolated from WT, APCmin/+or CAC mice. (b) COX2 expressed in the small intestine and the levels of IDEN PGE2 after anti-CD3 antibody treatment. (c) FACS analysis of CD4+Th17+cells in the duodenum after treatment with CD3-specific antibody with or without the COX2 inhibitors celecoxib or indomethacin. (d) ELISA analysis of IL-17A in supernatants from naive CD4+T cells under Th17+cell culture conditions in the presence of APC-IDENs with or without AH6809 or ONO-AE3–208. The data represent means±s.e.m. (n=5). *P<0.05,**P<0.005 (Student’st-test). Figure 7: APC-IDEN PGE2 plays a role in the accumulation of intestinal CD4 + Th17 + cells. ( a ) ELISA analysis of PGE2 in IDENs isolated from WT, APC min/+ or CAC mice. ( b ) COX2 expressed in the small intestine and the levels of IDEN PGE2 after anti-CD3 antibody treatment. ( c ) FACS analysis of CD4 + Th17 + cells in the duodenum after treatment with CD3-specific antibody with or without the COX2 inhibitors celecoxib or indomethacin. ( d ) ELISA analysis of IL-17A in supernatants from naive CD4 + T cells under Th17 + cell culture conditions in the presence of APC-IDENs with or without AH6809 or ONO-AE3–208. The data represent means±s.e.m. ( n =5). * P <0.05, ** P <0.005 (Student’s t -test). Full size image MyD88 regulates APC-IDEN recruitment and the activation of Th17 Previous studies [24] have suggested that the physical separation of microbiota from the intestinal surface is a restriction factor for immune activation, and perturbed spatial relationships between intestinal bacteria and hosts correlate with disease states such as inflammatory bowel disease (IBD). Our EM imaging data indicate that numerous tiny microvesicles observed in the intestinal lumen ( Fig. 8a , left panel) reside in the same compartment as intestinal bacteria ( Fig. 8a , right panel). Interestingly, CD63 + , an exosomal marker, was co-localized with 16S rRNA + in the outer mucosa layer ( Fig. 8b ). Confocal analysis showed a remarkable increase in the number of CD63 + IDENs that co-localized with 16S rRNA + bacteria in the colonic mucosa of APC min/+ mice compared with their co-housed wild-type littermates ( Fig. 8b ). CD63 + exosome/bacterial rRNA16 was also evident in isolated lymphoid follicles in APC Min/+ mice ( Fig. 8c ). In comparison with WT mice, APC Min/+ mice had greater quantities of CD63 + not only in the epithelial lumen ( Fig. 8d , top panels) but also in the lumen of the crypts ( Fig. 8d , bottom panels) and tumour tissue ( Fig. 8e ). Collectively, these data suggest that CD63 + IDENs co-localize with intestinal bacterial 16S rRNA + , and the depletion of the APC gene enhanced this co-localization and the number of CD63 + IDENs. 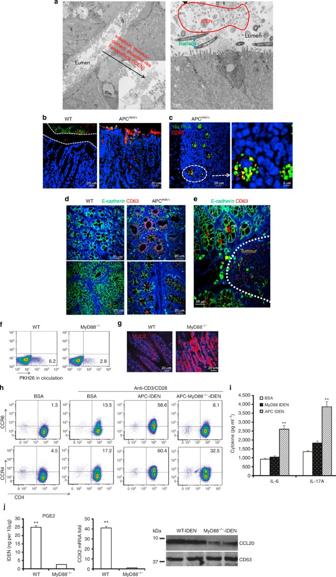Figure 8: MyD88 plays a role in the APC-IDEN-mediated induction of CCR6+CD4+Th17+cells. (a) Electron microscopy images of IDENs in the colons of wild-type B6 mice. (b,c) Confocal images of 16S RNA and CD63. CD63 (red) and bacterial 16S RNA (green) inhabiting loose mucous layers in colon tissue (b) and APCmin/+lymphoid follicles (c). (d,e) Confocal images of APCmin/+mouse CD63 in the epithelial lumen (d; top), the lumen of the crypts (d; bottom) and tumour tissue (e). (f,g) WT and MyD88−/−mice were treated with CD3-specific antibodies. FACS analysis of PKH26+cells in the peripheral blood after gavage with PKH26-labelled IDENs (f), confocal images of small intestine sections stained with a mucin-2-specific antibody (g). (h,i) Under Th17 cell culture conditions, naive CD4+T cells were cultured in the presence of BSA or IDENs. FACS analysis of the induced chemokine receptors (h) and ELISA of the production of cytokines (i). (j) ELISA analysis of IDEN PGE2 (Left panel) and real-time PCR analysis of COX2 (Middle panel) from the small intestine, and a western blot analysis of CCL20 in IDENs from mice treated with a CD3-specific antibody (Right panel). The data (i,j) represent means±s.e.m. (n=3).**P<0.01 (Student’st-test). Figure 8: MyD88 plays a role in the APC-IDEN-mediated induction of CCR6 + CD4 + Th17 + cells. ( a ) Electron microscopy images of IDENs in the colons of wild-type B6 mice. ( b , c ) Confocal images of 16S RNA and CD63. CD63 (red) and bacterial 16S RNA (green) inhabiting loose mucous layers in colon tissue ( b ) and APC min/+ lymphoid follicles ( c ). ( d , e ) Confocal images of APC min/+ mouse CD63 in the epithelial lumen ( d ; top), the lumen of the crypts ( d ; bottom) and tumour tissue ( e ). ( f , g ) WT and MyD88 −/− mice were treated with CD3-specific antibodies. FACS analysis of PKH26 + cells in the peripheral blood after gavage with PKH26-labelled IDENs ( f ), confocal images of small intestine sections stained with a mucin-2-specific antibody ( g ). ( h , i ) Under Th17 cell culture conditions, naive CD4 + T cells were cultured in the presence of BSA or IDENs. FACS analysis of the induced chemokine receptors ( h ) and ELISA of the production of cytokines ( i ). ( j ) ELISA analysis of IDEN PGE2 (Left panel) and real-time PCR analysis of COX2 (Middle panel) from the small intestine, and a western blot analysis of CCL20 in IDENs from mice treated with a CD3-specific antibody (Right panel). The data ( i , j ) represent means±s.e.m. ( n =3). ** P <0.01 (Student’s t -test). Full size image Next, we assessed the effects of intestinal bacteria on the IDEN-mediated induction of CD4 + Th17 + T cells. Oral transfer of IDENs from untreated APC Min/+ mice resulted in increased tumour size and number and percentage of IL17A-producing CD4 + T cells in the lamina propria of antibiotic-pretreated APC Min/+ mice. By contrast, untreated mice gavaged with IDENs from antibiotic-treated APC Min/+ mice failed to show an increase in the number or size of tumours, Th17 gene expression ( Supplementary Fig. S15a–15c ) or the expression of pSTAT3 and pERK ( Supplementary Fig. S15d ). Collectively, these data suggest that endogenous gut bacteria regulate the IDEN-mediated induction of Th17 cells and tumour growth. We then tested whether the activation of a TLR-MyD88 pathway affects the APC-IDEN-mediated induction of CCR6 + CD4 + Th17 + cells. In comparison with WT mice, MyD88 knockout led to a reduction in circulating PKH26 + IDEN + cells ( Fig. 8f ) and stronger intestinal Muc2 staining ( Fig. 8g ) in mice pretreated with anti-CD3 antibodies. FACS analysis further showed that IDENs from APC Min/+ /MyD88 −/− mice (APC/MyD88-IDEN) failed to induce the expression of chemokine receptors, particularly CCR6 and CCR4, on CD4 + T cells ( Fig. 8h ). The proinflammatory cytokines IL-17A and IL-6 were also decreased significantly in response to APC/MyD88-IDEN stimulation ( Fig. 8i ). Collectively, these data suggest that the MyD88-mediated pathway plays a role in increasing the quantity of circulating IDENs, and a higher number of circulating APC-IDENs leads to greater induction of CCR6 + CD4 + Th17 + cells. This conclusion is supported by the fact that CD3-specific antibody treatment failed to induce the accumulation of Th17 cells, diarrhea or liquid stools in the small intestines of MyD88 −/− or APC min/+ MyD88 −/− mice ( Supplementary Fig. S16a,S16b ). IDENs from MyD88 −/− mice pretreated with anti-CD3 treatment have much lower concentrations of COX2/PGE2 and CCL20 ( Fig. 8j ). Oral transfer of IDENs from MyD88 −/− APC min/+ mice fails to increase tumour number and size, recruitment of Th17 cells or the expression of pSTAT3 and pERK ( Supplementary Fig. S15a–15d ). In summary, these data suggest that the MyD88-mediated pathway plays a role in the APC-IDEN-mediated recruitment and activation of CCR6 + CD4 + Th17 + cells. The balance of Th17 and regulatory T cells in the gut is essential for maintaining gut homeostasis and preventing colon cancer and colon inflammatory-related diseases [25] . The results presented in this study suggest that a hierarchy of IDEN factors, each of which encompasses a distinct set of mechanisms, plays a role in the intestinal homeostasis of Th17 cells. First, IDEN CCL20+PGE2+ is an intestinal immune mediator that, at minimum, plays a role in both the recruitment and proliferation of Th17 cells. In colon tumour-bearing hosts, IDENs are more potent in their recruitment and proliferation of Th17 cells because of S1P-mediated overproduction of IDEN CCL20+PGE2+ . Second, unlike NT-BSPs, which induce regulatory T cells, ET-BSPs induce Th17 cells through the S1P-mediated overproduction of IDEN CCL20+PGE2+ . Finally, the induction of intestinal macrophage PGE2 by IDEN CCL20+PGE2+ further drives the overproduction of CD4 + CCR6 + IL17A + cells in colon tumour-bearing hosts. Furthermore, we found that intestinal bacterial genes encoding the B. fragilis toxin and PSA play a role in mediation of the balance of Th17 and regulatory T cells in the gut by BSPs. The significance of this finding lies in the well-known regulation of the balance of T reg/Th17 cells by gut bacteria. Whether gut bacteria-derived products such as BSPs participate in the modulation of this counterbalance has not been previously addressed; furthermore, if they do indeed participate, the molecular mechanism(s) underlying the counterbalance have yet to be defined. Our data suggest that bacteria are not required to be co-localized with host cells and bacteria-derived BSPs to direct and regulate this counterbalance. Unlike gut bacteria, BSPs can act over a long distance without causing infection, allowing bacteria to communicate with the host immune system by releasing BSPs. Another feature of BSPs is that they may provide a means for bacterial proteins and lipids such as sphingolipids [26] to be transported as a complex with other bacterial factors while being protected from degradation. Bacterial-derived factors such as S1P may also play a role in gut immunomodulation in collaboration with IDENs. Finally, S1P may contribute to the overproduction of IDEN CCL20+PGE2+S1P . S1P is known to promote tumour progression, and tumour cells produce much higher levels of S1P [27] than non-tumour cells. In this study, our data indicate that ET-BSPs are taken up by colon epithelial tumour cells, which leads to activation of the SphK1-mediated production of S1P. Our pharmacological inhibitor data suggest that S1P may promote the production of IDEN CCL20+PGE2+S1P . Numerous studies suggest that many different types of tumour cells secrete S1P and that S1P plays an important role in cancer progression [27] . The majority of the biological effects of S1P are known to be mediated via the activation of five specific G protein-coupled receptors (S1PR1–5) located on the cell surface [28] . Secreted S1P produced inside cells by sphingosine kinases can then signal through these receptors in an autocrine, paracrine and/or endocrine manner, which is termed the ‘inside-out signalling’ of S1P. A major current topic in S1P biology is how S1P is released from S1P producer cells. Because S1P possesses a polar head group, the S1P that is generated inside the cells cannot freely pass through the cell plasma membrane. Our study indicates that exosomes can be used as an S1P delivery vehicle for intercellular communication. In addition to the fact that intestinal exosome S1P regulates Th17 activity, other immune cells such as innate lymphoid cells also play a critical role in gut homeostasis [29] , [30] , [31] , [32] . Our findings will open up new avenues for determining whether intestinal exosome S1P regulates other immune cells, such as innate lymphoid cells, in gut homeostasis. It is conceivable that the transient induction of IDEN CCL20+PGE2+S1P+ is beneficial for cleaning up infectious agents, whereas the persistent release of IDEN CCL20+PGE2+S1P+ may cause chronic inflammation that generally promotes tumour progression [9] , [33] . IDEN-producing cells, that is, mouse intestinal epithelial cells, which are renewed every 4–5 days, have a limited lifespan and are likely to be crucial for gut homeostasis [34] . Intestinal epithelial cells exposed to pathogenic secreted particles (SPs) can induce appropriate mucosal immune responses, but the survival of intestinal epithelial cells containing pathogenic SPs is limited. Therefore, the pathogenic SP-mediated induction of IDEN CCL20+PGE2+S1P is terminated as a result of intestinal epithelial self-renewal. However, if IDEN-producing cells are transformed into colon tumour cells, the transformed cells could continuously release IDENs with higher levels of CCL20 + PGE2 + S1P + , which could drive the recruitment and induction of Th17 cells. Because many different types of tumour cells have been reported to release high levels of S1P [27] , [35] , it is conceivable that these tumour cells could release CCL20 + PGE2 + S1P + exosomes and mediate both the induction and recruitment of Th17 cells without ET-BSPs. The findings in our mouse model studies are directly translatable to human colon cancer. S1P and PGE2 levels are unregulated in human colon cancer patients [36] . S1P and PGE2 may therefore be promising targets for effective specific therapies. Because the free forms of S1P and PGE2 are unstable, one potential strategy would be to develop a method to accelerate S1P degradation by preventing S1P and PGE2 from associating with intestinal exosomes. On the basis of this study, we also speculate that two subsets of commensal bacteria SPs may coexist in the gut: one that induces Th17 cells and one that induces regulatory T cells. It has been reported that the phagocytosis of apoptotic cells in the absence of microbial signals induces the differentiation of regulatory T cells, whereas the phagocytosis of infected apoptotic cells induces Th17-cell differentiation [37] . Interestingly, the immunosuppressive nature of infected cell clearance coexists with the inflammatory nature of infection [37] . Commensal bacteria SPs are probably passing constantly through the lumen and being taken up by intestinal epithelial cells to release tolerogenic IDENs to induce regulatory T cells. Th17 cells predominantly recruit to the gut, and both Th17 cells and regulatory T cells are required for maintaining gut homeostasis, but whether there is also a subset of non-pathogenic SPs that regulate the immunogenic IDEN-mediated induction of Th17 remains unknown. Therefore, our findings warrant further research to determine whether two subsets of SPs are released from commensal bacteria: one regulating the tolerogenic IDEN-mediated production of regulatory T cells and other regulating immunogenic IDEN-mediated Th17-cell production. Dysregulation of this balance may lead to diseases such as colon cancer. Our data suggest that WT-IDENs may suppress CCL20 and other proinflammatory cytokines that are expressed in bacterial lysate-stimulated macrophages. Data published by other research groups [26] suggest that Bacteroides produce α-galactosylceramide, which regulates NKT activity. Our previously published data [4] , [5] also suggest that WT-IDENs suppress liver NKT-cell activation. We have not addressed in this study whether intestinal bacterial-derived factors incorporated into IDENs play a role in IDEN-mediated intestinal Th17 homeostasis, but we have provided a foundation for the future study of this topic. Animals and treatments C57BL/6J, Rag1 −/− , CCR6 −/− , OT-II and APC Min/+ mice on C57BL/6 background were obtained from Jackson Laboratories. Myd88 −/− mice on C57BL/6 background were kindly provided by S. Akira (Osaka Univ., Osaka, Japan), and were crossed to APC Min/+ mice. All animal procedures were approved by the University of Louisville Institutional Animal Care and Use Committee. Mouse models of colon cancer (1) APC Min/+ mice carrying a mutation in Apc gene that mimics familial adenomatous polyposis and the majority of sporadic colon cancers and (2) colitis associated colon cancer (CAC) models were induced by azoxymethane (AOM) treatment followed by dextran sodium sulfate (DSS). AOM was injected intraperitoneally into 6- to 8-week-old male mice at 15 mg kg −1 . One week after the injection, the mice were exposed to three cycles of 1 week of 2.5% DSS (molecular weight 36,000–50,000; MP Biomedicals) in the drinking water followed by 2 weeks of normal water regimen. Colitis was induced using a 2.5% solution of DSS that was provided as drinking water to mice (18–25 g, 6 weeks old, male) for 10–12 days. (3) In the third model, mice had an orthotopic colonic submucosal implantation of colon cancer cells. Seven-week-old female mice were anaesthetized using Ketamine/Xylazine and submucosal injections were accomplished using a murine colonoscopy system, which consisted of a miniature endoscope, a xenon light source, a triple chip camera and an air pump (Karl Storz, Tuttlingen, Germany). In brief, 10 μl (1 × 10 5 ) of MC38 tumour cells with or without ectopic luciferase expression were inserted through a Luer lock (Söllner, GmbH) stainless needle screwed on the working channel of the scope. The scope was then inserted into the mouse colon and the needle was brought through the working channel to the scope’s front. The injection was performed by a very gentle sub-mucosal penetration with the open side of the bevel heading up at a flat angle. Isolation and purification of IDENs Mice were euthanized and the intestine removed. The luminal contents of the intestine were removed by gently flushing the intestine with 10 ml of ice-cold PBS. The intestine was then opened longitudinally, the mucous collected by mild physical separation using round forceps, soaked in PBS, then agitated on a rotator at 70 r.p.m. min −1 for 15 min and centrifuged at 500 × g for 15 min at 4 °C. The supernatant was then followed by differential centrifugation and sucrose gradient centrifugation to isolate and purify the exosomes using a previously described protocol [38] . Protein concentration was determined using the Bio-Rad Protein Quantitation Assay kit with bovine serum albumin as a standard. Each lot of IDENs used for this study was also FACS analysed for CD63, an exosomal marker, and A33, a marker of intestinal epithelial cells. Exosomes used in this study were always more than 90% of CD63 + A33 + IDENs. Adoptive transfer of IDENs or exosomes Adoptive transfer of various IDENs (250 μg in PBS) was performed once every 3 days for 8 weeks by oral administration in APC Min/+ mice at 6 weeks of age with/without antibiotic treatment. IDENs (APC-IDENs) were isolated from APC Min/+ mice at 4 months of age. IDENs (CAC-IDENs) (250 μg) were isolated from CAC mice 3–4 months after AOM plus DSS administration. CAC-IDENs were intra-rectally transferred into AOM-treated mice after the first DSS cycle. IDENs were delivered through a 1.2-mm-diameter polyurethane catheter (Access Technologies) for 8 weeks. Mice were euthanized at 3 months of age and polyps were counted using a stereomicroscope. Tumour exosomes (250 μg) derived from MC38 cells treated by ET-BSP or NT-BSP were transferred into tumour-bearing mice or naive mice by colonic submucosal injection every 2 days for 18 days. Colon sections were fixed in formalin or snap frozen. In some experiments, polyps were harvested individually and frozen in liquid nitrogen. Antibiotic or antibody treatment Mice were given the following antibiotics in autoclaved drinking water: ampicillin (1 g l −1 ; Sigma), vancomycin (500 mg l −1 ; Henry Schein) neomycin sulfate (1 g l −1 ; Sigma) and metronidazole (1 g l −1 ; Sigma; solubilized with 15 ml of 0.1 N acetic acid per litre). Fresh antibiotics were supplied every 3 days. Mice were kept on antibiotics for the indicated time and killed for tumour and tissue analysis. Mice were administered IDENs resuspended in PBS by gavage or intravenous injection as described previously [39] . In some experiments, neutralizing antibody (200 μg per mouse) for IL-17A (MAB421 R&D Systems) or control IgG was injected once every week for 8 weeks. Apc Min/+ and Apc Min/+ /MyD88 −/− littermates were euthanized at 3−4 months of age or when the first signs of morbidity appeared. The intestinal tract was removed immediately after euthanasia. The small intestine and colon were examined, and tumours were counted and measured using a stereomicroscope. Most polyps were adenomas, identified by their appearance as grossly visible, preinvasive lesions that were common in the small intestine of APC Min/+ mice. Colonic lesions that displayed a focally invasive phenotype were categorized as tumours. Five-μm sections of paraffin-embedded specimens were cut and stained with H&E for histology analyses. Induction of colitis T-cell mediated colitis was induced in Rag1 −/− mice by adoptively transferring CD4 + CD25 − CD62L + T cells sorted using a FACSAria II flow cytometer (BD Biosciences). The Rag1 −/− recipients were given 5 × 10 5 CD4 + CD25 − CD62L + T cells via intraperitoneal injection, and were euthanized at 6–7 weeks after transfer. For the adoptive transfer of IDEN experiment, some recipient mice also received by oral administration 250 μg of WT-IDENs or APC-IDENs once every 3 days for 6 weeks after the transfer of CD4 + CD25 − CD62L + T cells. Colitis was also induced in C57BL/6J mice by the addition of 2.5% (wt/vol) DSS (36–50 KD molecular weight, MP Biomedicals, OH) in their drinking water. Beginning at day −10 of DSS treatment, mice were orally treated with PBS, NT-BSP (200 μg) or ET-BSP (200 μg) every other day for 20 days. DSS solution was freshly prepared every other day. Body weight and physical activity were monitored daily. Flow cytometry For analysis of surface markers, cells were stained in PBS containing 2% (wt/vol) BSA. Intracellular staining of the transcription factors Foxp3 was performed using the Foxp3 Fix/Perm Buffer Set (Biolegend). For detection of intracellular cytokines, cells were first stimulated for 4 h with 50 ng ml −1 PMA and 1 μg ml −1 ionomycin in the presence of Brefeldin A (All obtained from Sigma), followed by staining for surface markers. Cells were then fixed and permeabilized using the Foxp3 Fix/Perm Buffer Set (Biolegend) and stained for intracellular cytokines. The following antibodies were used at a dilution of 1/200–1/600: PerCP-Cy5.5, PE-, FITC- or APC-labeled anti-IL-17 (TC11–18H10.1), PE- or APC-labelled anti-IL-10 (JES5–16E3), PE-labelled anti-Foxp3 (FJK-16 s, eBioscience), PE-, FITC- or APC-labelled anti-CCR6 (29-2L17), PE-, FITC- or APC-labelled anti-CD4 (RM4–5), PE-Cy7-labelled anti-CD3 (145-2C11), APC- or PE-Cy7-labelled anti-IFN (XMG1.2), FITC-, PerCP-Cy5.5 or Pacific Blue-labelled anti-CD45 (30-F11), PE-anti-CCR4 (2G12), PE- or FITC-labelled anti-CCR9 (CW-1.2). All antibodies were obtained from Biolegend unless otherwise noted. Flow cytometry data were acquired on a 5-colour FACScan (Becton Dickinson), and analysed using FlowJo software (Treestar). Cell sorting was performed using a FACSAria II. Histology and immunohistochemistry Tissue specimens were fixed in 10% formalin, dehydrated and then embedded in paraffin. Tissue samples were cut at 5 μm thicknesses and stained with haematoxylin and eosin. For immunofluorescence analysis, tissue sections were subjected to antigen retrieval by boiling the slides in Antigen Unmasking Solution (Vector Laboratories) for 10 min according to instructions. Sections were then blocked for 1 h at 22 °C with 5% BSA in PBS and incubated overnight at 4 °C with the primary antibodies (rabbit polyclonal Ki67, phospho-Stat3 Tyr705 and phospho-Erk antibody from Cell Signaling used at a dilution of 1/100, and rat polyclonal CD63, Muc2 from AbCam (Cambridge, MA), rabbit polyclonal CD63, Jam-a from Santa Cruz Biotechnology (Santa Cruz, CA) used at a dilution of 1/50, CD11b and E-Cadherin were gained from BD Bioscience (San Jose, CA) and used at a dilution of 1/100. Primary antibodies were detected by Alexa Fluor 488, 594 or 647 conjugated goat anti-mouse, anti-rabbit IgG and anti-rat (1:600, Invitrogen), respectively. Tissues were counterstained with DAPI and images were captured on a Zeiss LSM 510 confocal microscope equipped with a digital image analysis system (Pixera). For immunofluorescence analysis of macrophages, OCT (Sakura Finetek)-embedded tissue cryosections (9 μm-thick) were stained by F4/80 (BM8, ebioscience). Western blot analysis Exosomes or cells were disrupted in lysis buffer containing 1% Triton X-100, 0.1% SDS, 150 mM NaCl, 50 mM Tris-HCl, 1 mM EDTA, 1 mM EGTA, 5 mM sodium molybdate and 20 mM phenylphosphate with protease and phosphatase inhibitors (1 mM PMSF, 10 μg ml −1 aprotinin, 20 μg ml −1 leupeptin, 20 μg ml −1 pepstatin A, 50 mM NaF and 1 mM sodium orthovanadate) for 30 min on ice. The samples were centrifuged (16,000 × g , 10 min, 4 °C) and the resulting supernatants transferred to fresh tubes. Protein lysates were quantitated using a Bio-Rad protein kit (Bio-Rad) and 50 μg of exosomal lysates were separated on 10% SDS polyacrylamide gels and transferred to a nitrocellulose membrane. Rabbit anti-Stat3 (727), p-Stat3 (705), STAT3 and actin were purchased from Cell Signaling Technology (Danvers, MA) and used at a dilution of 1/1,000. Anti-CCL20 was purchased from Biorbyt (San Francisco,CA) and used at a dilution of 1/1,000. Membranes were probed with specific antibodies and protein quantity visualized using an Odyssey instrument (Li-CoR Bioscience). Images have been cropped for presentation. Full-size images are presented in the Supplementary Material . RNA extraction and PCR Total RNA was isolated from the distal small intestine, lamina propria lymphocytes (LPL) or MA38 tumour cells using the Qiagen RNeasy RNA isolation Kit and was used to synthesize cDNA. RNA (1 μg) was reverse-transcribed with Superscript III and random primers (Invitrogen). For quantitation of genes of interest, cDNA samples were amplified in a CFX96 Realtime System (Bio-Rad Laboratories, Hercules, CA, USA) and SYBR Green Master Mix (Invitrogen) and specific primers ( Supplementary Table 1 ) according to the manufacturer’s instructions. Fold changes in mRNA expression between treatments and controls were determined by the δCT method as described [40] . Differences between groups were determined using a two-sided Student’s t -test and one-way ANOVA. Error bars on plots represent±s.e., unless otherwise noted. The data were normalized to a GAPDH reference. All primers were purchased from Eurofins MWG Operon. Fluorescence in situ hybridization Intestinal tissues were prepared for FISH analysis by fixation in Carnoy’s fixative (Electron Microscopy Sciences, Hatfield, PA). Two 30-minute washes in dry methanol were followed by two 20-minute washes in absolute ethanol. Before paraffin embedding and sectioning, the fixed tissue was incubated twice in xylene for 15 min. Tissues were sectioned at a thickness of 5 μm and FISH analysis was performed using the EUB338 probe (GCTGCCTCCCGTAGGAGT) labelled with Alexa488, against 16S rRNAs from most bacteria. The nonsense probe Non338 (ACTCCTACGGGAGGCAGC) was used to test for nonspecific binding of oligonucleotide probes. Hybridizations were carried out and tissues were visualized using a Zeiss LSM 510 confocal microscope. Bacterial strains and growth conditions Non-enterotoxigenic Bacteroides fragilis strain NCTC9343 and enterotoxigenic Bacteroides fragilis strain (20656-2-1) were obtained from the American Type Culture Collection. Nontoxigenic wild-type B. fragilis (WT-NTBF) overexpressing BFT (γETBF; BFT-2 ) and WT-NTBF overexpressing a biologically inactive mutated BFT (ΔBFT; bft-2 H352Y) were kindly provided by Dr Sears [41] . Wild-type NCTC9343 with mutant polysaccharide A (PSA) was kindly provided by Dr Comstock [42] , [43] . Bacteroides fragilis were cultured either in brain heart infusion (BHI) broth (BD Biosciences) or in 1 l of basal PYG medium containing 5 g glucose, 1% FBS, 0.5 mg haemin, and 0.5 mg ml −1 vitamin K, 0.5 g L -cysteine, 5 g potassium phosphate. Cultures were grown at 37 °C under anaerobic conditions. Pharmacological agents IDEN lipids were extracted according to Bligh and Dyer [44] in chloroform/methanol/water (2.5:2.5:2.1, v/v/v). Lipids for treatment of cells were dried under nitrogen and sonicated in PBS at pH 7.4 and 0.05% (vol/vol) Tween-20 before use. PGE 2 , Butaprost, misoprostol, sulprostone and PGE 2 ELISA kits were obtained from Cayman Chemical. EP4 agonists (ONO-AE1–329), EP1 antagonist (ONO-8713), EP3 antagonist (ONO-AE3–240) and EP4 antagonist (ONO-AE3–208) were kind gifts from Ono Pharmaceutical Company. SK1-I and W146 were obtained from Sigma. BSP purification and labelling BSP was isolated and purified from cultured bacteria. B. fragilis was grown in PYG media to early stationary phase. B. fragilis bacteria were removed by pelleting (2000 × g , 20 min; 10,000 × g , 1 h). BSP were then recovered from the bacteria-free culture supernatant by centrifugation (100,000 × g , 1.5 h), purified by sucrose gradient centrifugation using a previously described protocol [38] , and washed with PBS by centrifugation at 100,000 × g for 1 h. The pellet was resuspended in PBS, and stored at −80 °C until used. PKH26-labelled BSP were prepared as previously described [4] . Isolation of LPLs and flow cytometry analysis The method used for isolation of LPLs has been previously described [45] . In brief, fat tissues and PPs were removed from small intestine. The intestine was open and cut in pieces 1-cm long and incubated in an HBSS solution containing 5 mM EDTA and 10 mM Hepes) for 30 min at 37 °C with slow rotation (180 r.p.m. min −1 ). Pieces were then further cut and incubated in an HBSS solution containing 0.5 mg ml −1 DNase I (Roche) and 1 mg ml −1 Collagenase type IV (Worthington). Finally, the solution containing digested tissue was passed through a 100-μm cell strainer and LPLs were recovered at the interface of the 40 and 80% Percoll (GE Healthcare) solutions. For flow cytometry analysis, the cells were labelled using standard procedures [46] . Cells were analysed by flow cytometry using a FACScan (BD Biosciences protocol; BD Pharmingen). In some experiments, stained cells were sorted to purify indicated populations on a BD FACS Aria III. Histogram analysis was performed using FlowJo software (Treestar, Ashland, OR). ELISA IL-6, IL-10 and IL-17 in culture supernatants were quantified using ELISA kits (eBioscience). For PGE2 assay, lipids were extracted from exosomes and IDENs in 70% cold ethanol, 30% monobasic sodium phosphate (0.1 M), pH 4.0, followed by shaking incubation for 30 min at 24 °C. Homogenates were centrifuged at 1,000 × g for 10 min. Triplicate aliquots of supernatants were dried under nitrogen, and the PGE2 concentration was determined by ELISA (Cayman Chemical). Cell cultures For IDEN-mediated Th17 differentiation, naive T cells were cultured for 5 days with anti-CD3 (5 μg ml −1 , 2C11, Bio X cell), anti-CD3, anti-CD28 (2 μg ml −1 , 37.51; Bio X Cell), IL-6 (20 ng ml −1 ), TGF-β1 (2 ng ml −1 ; R&D Systems), anti-IL-4 (10 μg ml −1 ), anti-IFN-γ (10 μg ml −1 ) and IL-23 (20 ng ml −1 ) in the presence of IDENs (50 μg ml −1 ), followed by stimulation with PMA and ionomycin in the presence of GolgiStop. Intracellular cytokine production and chemokine receptor expression on CD4 + T cells were then determined by flow cytometry. For colonic macrophages, T-cell co-cultures, 5 × 10 4 macrophages and 2.5 × 10 5 OT-II T cells were mixed in the presence of cognate peptide (5 μg ml −1 ; OVA) and/or IDENs (50 μg ml −1 ). After 4 days of culture, live T cells were collected and stimulated with PMA (phorbol 12-myristate 13-acetate, 50 ng ml −1 ) and ionomycin (1 μg ml −1 Sigma) plus brefeldin A (10 μg ml −1 Sigma) for intracellular cytokine staining or for mRNA analysis. To study the activity of BSP on tumour cells, the colon cancer cell line MC38 was acquired from the American Type Culture Collection and cultured as recommended. MC38 cells were cultured with BSP (50 μg ml −1 ) in the absence or presence of 5 μM SK1-I for 48 h, exosomes were prepared according to a previously described protocol [47] . In some experiments, MC38 cells were treated with S1P (100 nM). mRNA were assessed by RT-PCR or supernatants were used for cytokine measurement by ELISA. Chemotaxis assay Cultured CD4 + T cells from C57BL/6 mice or CCR6-KO mice were resuspended in complete RPMI-1640 medium and were loaded into collagen-coated Transwell devices (pore size, 5 mm; 3421; Corning) placed in 24-well plates containing medium alone or medium supplemented with 50 μg ml −1 WT-IDEN or APC-IDEN. After plates had incubated at 37 °C for 4 h, cells that had migrated were collected, counted and stained with mAb to determine the number of migrated CD4 + T cells by flow cytometry. The ratio of the number of CD4 + T cells that migrated in the presence of IDENs to the number of cells that migrated to control media was calculated and is presented as the percentage of migrated cells relative to the input. Anti-CD3 antibody treatment Mice were injected with anti-CD3 (20 μg per mouse, Bio X cell, 145 2C11) [1] intraperitoneally three times at an interval of 2 days between injections and killed 4 h after the final injection. In some experiments, mice were co-treated with COX2 inhibitor indomethacin (3 mg kg −1 of body weight) or celecoxib (15 mg kg −1 of body weight) by intraperitoneal injection. Sphingolipid analysis Ceramide species, sphingosine and S1P from IDEN and tumour exosmes were collected and analysed using a S1P ELISA kit (Mybiosource, #MBS094198) or with LC-MS/MS by the Lipidomics Shared Resource (Medical University of South Carolina), as previously described [48] . In brief, calibration curves were constructed by plotting peak area ratios of synthetic standards corresponding to each target analyte with respect to the appropriate internal standard. The target analyte peak areas from the samples were similarly normalized to their respective internal standard and then compared with the calibration curves using a linear regression model. Results were normalized to total protein levels Statistical analysis Multiple comparisons were analysed by one-way ANOVA and Fisher’s protected least significant difference test. A t -test was used to compare the means of two groups. P values of <0.05 were considered to be statistically significant. How to cite this article: Deng, Z. et al. Enterobacteria-secreted particles induce production of exosome-like S1P-containing particles by intestinal epithelium to drive Th17-mediated tumorigenesis. Nat. Commun. 6:6956 doi: 10.1038/ncomms7956 (2015).